IGF-1 promotes the development and cytotoxic activity of human NK cells Insulin-like growth factor 1 (IGF-1) is a critical regulator of many physiological functions, ranging from longevity to immunity. However, little is known about the role of IGF-1 in natural killer cell development and function. Here, we identify an essential role for IGF-1 in the positive regulation of human natural killer cell development and cytotoxicity. Specifically, we show that human natural killer cells have the ability to produce IGF-1 and that differential endogenous IGF-1 expression leads to disparate cytotoxicity in human primary natural killer cells. Moreover, miR-483-3p is identified as a critical regulator of IGF-1 expression in natural killer cells. Overexpression of miR-483-3p has an effect similar to IGF-1 blockade and decreased natural killer cell cytotoxicity, whereas inhibition of miR-483-3p has the opposite effect, which is reversible with IGF-1 neutralizing antibody. These findings indicate that IGF-1 and miR-483-3p belong to a new class of natural killer cell functional modulators and strengthen the prominent role of IGF-1 in innate immunity. Natural killer (NK) cells represent a distinct lymphocyte subset with a central role in innate immunity, and accumulating evidence in mice and humans suggests that NK cells serve important functions in influencing the nature of the adaptive immune response [1] , [2] . The cytotoxic function of NK cells is crucial to many processes such as defending against pathogens and tumors [3] , [4] . The cytotoxic mechanisms of NK cell action are mediated predominantly via perforin and granzymes, which are essential effector molecules for NK cell cytotoxic activity [5] , [6] . Following granule exocytosis, perforin facilitates the delivery of granzymes into the cytosol of the target cell where they cleave numerous substrates, including caspases, resulting in the rapid induction of apoptosis [7] , [8] . Human NK cells can be classified into CD56 bright and CD56 dim subsets based on cell-surface CD56 density; these subsets differ in function, phenotype and tissue localization [9] . Low-density CD56 (CD56 dim ) subsets occupy more than 90% of peripheral blood NK (pNK) cells and express high levels of perforin, CD16 and killer Ig-like receptors. The subset of CD56 bright NK cells, which are rare in blood but predominate in lymph nodes, inflamed tissues and deciduas [10] , [11] , [12] , express low levels of perforin and killer Ig-like receptor [13] . In contrast, CD56 dim cells are highly cytotoxic and preferentially produce cytokines after recognition of target cells [14] , [15] . However, the mechanism behind these differences in human NK cell cytotoxic activity is not well understood. In vitro , human NK cells can differentiate from bone marrow- or cord blood-derived hematopoietic progenitor cells in the presence of cytokines alone. Furthermore, a number of different cytokine combinations have been tested for their ability to support the proliferation and differentiation of human CD34 + hematopoietic stem cells (HSCs) into mature NK cells. A cytokine that has not been extensively studied in this regard is IGF-1. IGF-1, also known as somatomedin C, is one of the main endocrine mediators of growth and development under physiological conditions [16] . In addition to this important function, IGF-1 also has a prominent role in the regulation of immunity and inflammation. Increasing evidence suggests that IGF-1 also regulates hematopoiesis and direct effector functions of cells of the innate and acquired immune systems. IGF-1 has complex regulatory functions in adult human hematopoietic progenitor cells and can stimulate the proliferation of both myeloid and erythroid progenitors through its interactions with IGF-1 receptor (IGF-1R) [17] , [18] . Moreover, IGF-1 regulates diverse aspects of T-cell, B-cell and monocyte function through its interactions with IGF-1R. Nearly all cells of the immune system including T and B lymphocytes [19] , peripheral blood mononuclear cells (PBMCs) [20] and NK cells [21] express IGF-1R and are therefore susceptible to the effects of IGF-1. However, very little is known about the role of IGF-1 in NK cell development and function. Oligonucleotide microarray data indicate that pNK cells and CD56 bright uterine decidual NK (dNK) cells differ in their patterns of gene expression [12] . Subsequent work has shown differential capabilities of CD56 dim and CD56 bright NK populations with respect to the secretion of soluble factors. In particular, IGF-1 was preferentially produced by CD56 dim NK cells [22] . However, the molecular mechanism underlying the regulation of IGF-1 expression in human NK cells remains unclear. Recently, a group of noncoding microRNAs (miRNAs) binding to the 3′ untranslated region (UTR) of target mRNAs (which results in degradation of the target mRNAs or translational repression of the encoded proteins [23] ) was shown to have a critical role in controlling NK cell homoeostasis, activation and effector function, in addition to regulating diverse aspects of NK cell biology [24] , [25] , [26] , [27] , [28] , [29] . We hypothesized that the IGF-1 gene may be targeted for downregulation by miRNAs in CD56 bright NK cells to allow for attenuation of the cytotoxicity. Here we demonstrate that IGF-1 promotes NK cell development from human CD34 + HSCs and that IGF-1 increases the cytotoxic potential of both CD34 + HSC-derived NK cells and CD56 bright uterine dNK cells. Specifically, we provide evidence that endogenous IGF-1 is regulated by miR-483-3p in human NK cells, which then contributes to NK cell cytotoxicity. Moreover, in dNK cells isolated from human patients who underwent spontaneous abortions, IGF-1 production was upregulated, which correlated with increased cytotoxicity and lower miR-483-3p expression. Collectively, our results suggest that IGF-1 is a significant modulator of NK cell development and function and that miR-483-3p has a role in regulating NK cell cytotoxicity. IGF-1 promotes the development of human NK cells IGF-1 has been demonstrated to promote T-cell development in the thymus and early B-cell development in the bone marrow [30] . It also has a costimulatory effect on the in vitro proliferation of committed progenitors derived from human umbilical cord blood (UCB) CD34 + cells [31] . However, the potential role of IGF-1 in NK cell development is unknown. To investigate a potential role for IGF-1 in human NK cell development, cultured UCB/CD34 + HSCs ( Supplementary Fig. S1a ) were maintained with Flt3-L and stem cell factor (SCF) in the presence of either interleukin 15 (IL-15), IGF-1 or a combination of both cytokines for up to 4 weeks. We found that either IL-15 alone or, even more dramatically, the combination of IL-15 and IGF-1 activated the proliferation of CD34 + cells ( Fig. 1a ). Proliferation was increased substantially in CD34 + cell cultures containing both IL-15 and IGF-1 ( Fig. 1b ). Moreover, when SCF/Flt3-L/IL-15-containing media was supplemented with IGF-1, a significant increase was observed in the percentages and absolute cell numbers of CD56 + NK cells ( Fig. 1c ), suggesting that IGF-1 contributes to the development of NK subsets. We also observed that other factors (such as IL-7, IL-12 or IGF-2) slightly enhanced NK cell expansion ( Supplementary Fig. S1b,c ). We further investigated how IGF-1 promoted NK cell development. Specific transcription factors ‘program’ the developmental pathway from HSCs towards lineage-restricted differentiation [32] . NFIL3 (also known as E4BP4), a basic leucine zipper transcription factor, is a critical regulator of NK cell development through its induction of the transcriptional inhibitor Id2 (refs 33 , 34 ). Hence, we assessed how IGF-1 affects expression levels of mRNA encoding the NK-associated transcription factors NFIL3 and ID2. The provision of IGF-1 to CD34 + cells was associated with upregulated mRNA signals for NFIL3 and ID2 ( Fig. 1e ), which correlated with the increased NK cell production. 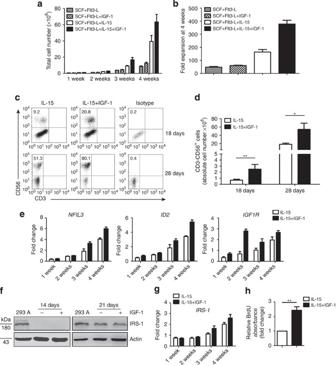Figure 1: IGF-1 induces the differentiation and expansion of human UCB/CD34+cells into NK cells. (a) Total number of viable cells differentiated from CD34+cells by various cytokine combinations, as counted for up to 4 weeks. (b) Fold expansion of UCB CD34+cells after 4 weeks of culture with either of the cytokine combinations. (c) Representative flow-cytometry analysis of the relative ratio of NK cells cultured with either IL-15 or the combination of IL-15 and IGF-1 at the indicated time. (d) The absolute number of CD56+CD3−NK cells analysed inc. (e)NFIL3, ID2andIGF-1Rexpression in cytokine-differentiated CD34+cells at the indicated time, as quantified by quantitative reverse transcription PCR (qRT–PCR). (f,g) Immunoblot analysis (f) and qRT–PCR analysis (g) of the expression of IRS-1 in CD34+HSCs cultured with IL-15 or the combination of IL-15 and IGF-1 at the indicated time. (h) Proliferation of CD34+HSCs cultured with IL-15 or the combination of IL-15 and IGF-1 at day 21 was measured by BrdU proliferation ELISA assay. Data are representative of three independent experiments (mean±s.e.m.). *P<0.05 and**P<0.01 (Student’st-test). Figure 1: IGF-1 induces the differentiation and expansion of human UCB/CD34 + cells into NK cells. ( a ) Total number of viable cells differentiated from CD34 + cells by various cytokine combinations, as counted for up to 4 weeks. ( b ) Fold expansion of UCB CD34 + cells after 4 weeks of culture with either of the cytokine combinations. ( c ) Representative flow-cytometry analysis of the relative ratio of NK cells cultured with either IL-15 or the combination of IL-15 and IGF-1 at the indicated time. ( d ) The absolute number of CD56 + CD3 − NK cells analysed in c . ( e ) NFIL3, ID2 and IGF-1R expression in cytokine-differentiated CD34 + cells at the indicated time, as quantified by quantitative reverse transcription PCR (qRT–PCR). ( f , g ) Immunoblot analysis ( f ) and qRT–PCR analysis ( g ) of the expression of IRS-1 in CD34 + HSCs cultured with IL-15 or the combination of IL-15 and IGF-1 at the indicated time. ( h ) Proliferation of CD34 + HSCs cultured with IL-15 or the combination of IL-15 and IGF-1 at day 21 was measured by BrdU proliferation ELISA assay. Data are representative of three independent experiments (mean±s.e.m.). * P <0.05 and ** P <0.01 (Student’s t -test). Full size image We also found that IGF-1 induced a significant increase in IGF-1R mRNA expression levels in human CD34 + -derived NK progenitors responsive to IL-15-induced differentiation at 2 weeks, which persisted until culture termination after 4 weeks ( Fig. 1e ). IGF-1/IGF-1R induces differentiation rather than proliferation when the cells do not express or underexpress insulin receptor substrate-1 (IRS-1), a docking protein for both IGF-1R and the insulin receptor that is known to send a mitogenic, anti-apoptotic and anti-differentiation signal [35] , [36] . To provide further mechanistic insight into the role of IGF-1/IGF-1R in NK cell development, we investigated the levels of IRS-1 in human CD34 + cells cultured with either IL-15 or the combination of IL-15 and IGF-1 at 14 or 21 days and compared it with the levels of IRS-1 in 293A cells, which usually expressed normal levels of IRS-1. CD34 + HSCs differentiated into NK cell precursors after being cultured in SCF/Flt3-L/IL-15-containing media with or without IGF-1 for 14 days. An important characteristic of these cells is that they do not express IRS-1 ( Fig. 1f ), Thus, IGF-1 likely induces the cells to differentiate. This finding is in agreement with previous studies demonstrating that IRS-1 levels are low or even absent in differentiating cells [37] . Although NK cell precursors differentiated into CD3 − CD56 + NK cells after stimulation with IL-15 or IL-15 plus IGF-1 for an additional 7 days (a total of 21 days), in those cells that express IRS-1 ( Fig. 1f ), proliferation prevails, and this was confirmed in follow-up studies using a bromodeoxyuridine (BrdU) cell-proliferation assay ( Fig. 1h ). Based on these results, it is likely that IGF-1/IGF-IR does indeed activate both differentiation and proliferation programs. Exogenous IGF-1 enhances NK cell cytotoxicity We next characterized the expression of an array of potentially informative activation antigens on cytokine-modulated CD34 + cells. We examined the expression of NKp30, NKp44, NKG2D and CD69 in UCB/CD34 + -derived NK cells cultured for 28 days in the presence or absence of IGF-1. No statistically significant differences could be observed for most of the examined receptors. However, the presence of IGF-1 induced the upregulation of CD69 on human NK cells from UCB CD34 + HSCs ( Supplementary Fig. S2 ). CD69 is a functional triggering molecule on activated NK cells and is one of the earliest expressed cell-surface activation markers that is capable of mediating NK cell cytotoxicity. Thus, we postulated that IGF-1 may improve NK cell cytotoxic activity and that other molecules may be implicated in the increased cytotoxic potential of NK cells derived from UCB/CD34 + cells in the presence of IGF-1. The expression of CD107a on the cell membrane correlates with NK cell killing activity [38] . We observed that the presence of IGF-1 significantly increased CD107a release in human CD34 + -derived CD56 + NK cells compared with that of CD56 + effectors derived from the same CD34 + population in the presence of SCF, Flt3-L and IL-15 alone ( Fig. 2a ). In support of this increased NK cytotoxic potential, the expression of the NK cytotoxic effector-associated gene perforin, as determined by flow-cytometric analysis or quantitative real-time PCR analysis in CD56 + NK cells, was also significantly increased in the above IGF-1-induced CD34 + -derived NK cells compared with the cells without IGF-1 ( Fig. 2a ). Moreover, the provision of IL-15 and IGF-1 to CD34 + cells was associated with upregulated mRNA signals for PRF1 (which encodes perforin), GzmB (which encodes Granzyme B) and IFNG (which encodes interferon-γ (IFN-γ)) ( Fig. 2b ). These results indicate that IGF-1 is capable of increasing the cytotoxic potential of NK cells derived from human CD34 + cells. 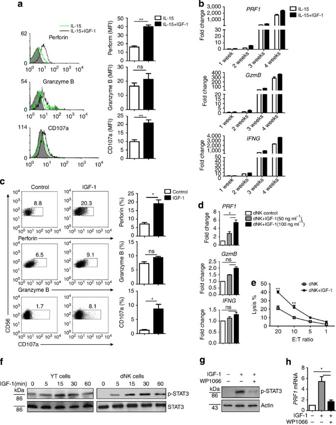Figure 2: IGF-1 induces increased human NK cytotoxic potential. (a) Flow cytometry for perforin, Granzyme B and CD107a expression in human UCB-CD34+-derived CD3−CD56+NK cells cultured for 28 days in the presence (black line) or absence (green line) of IGF-1. The grey histogram represents the isotype-matched negative controls. The graphs show the mean fluorescence intensity (MFI) of perforin, Granzyme B and CD107a expression in the above cells. (b)PRF1,GzmBandIFNGexpression in cytokine-differentiated CD34+cells at the indicated time in the presence or absence of IGF-1, as quantified by quantitative reverse transcription PCR (qRT–PCR). (c) Flow cytometry for perforin, Granzyme B and CD107a expression in purified human uterine dNK cells cultured for 24 h with and without IGF-1 (control). The graphs show the average relative frequency of all perforin+, CD107a+or Granzyme B+dNK cells as above. (d) RelativePRF1,GzmBandIFNGexpression levels in purified human uterine dNK cells cultured for 24 h with IGF-1 at the indicated concentrations, as quantified by qRT–PCR. (e) Chromium-release assay using51Cr-labelled K562 cells co-cultured with untreated dNK cells (open squares) or dNK cells from the same preparation incubated for 24 h with IGF-1 (100 ng ml−1) in RPMI medium 1640 plus 10% fetal calf serum (filled squares) at various effector-to-target (E:T) ratios. (f) YT and primary dNK cells were deprived of serum for 4 h and were then stimulated with 100 ng ml−1IGF-1 for 0, 5, 15, 30 and 60 min, separately. The cells were washed by PBS and collected. The whole-cell extracts were prepared for western blotting to examine STAT3 and phosphorylation of STAT3. (g,h) The dNK cells were pretreated with WP1066 (100 μM) for 30 min or left untreated, followed by treatment with or without IGF-1 (100 ng ml−1) for 24 h. The presence of phospho-STAT3 was probed by western blot analysis (g), and perforin gene expression was quantified by qRT–PCR (h). Data are representative of three independent experiments (mean±s.e.m.). *P<0.05 and**P<0.01 (Student’st-test). ns, not significant. Figure 2: IGF-1 induces increased human NK cytotoxic potential. ( a ) Flow cytometry for perforin, Granzyme B and CD107a expression in human UCB-CD34 + -derived CD3 − CD56 + NK cells cultured for 28 days in the presence (black line) or absence (green line) of IGF-1. The grey histogram represents the isotype-matched negative controls. The graphs show the mean fluorescence intensity (MFI) of perforin, Granzyme B and CD107a expression in the above cells. ( b ) PRF1 , GzmB and IFNG expression in cytokine-differentiated CD34 + cells at the indicated time in the presence or absence of IGF-1, as quantified by quantitative reverse transcription PCR (qRT–PCR). ( c ) Flow cytometry for perforin, Granzyme B and CD107a expression in purified human uterine dNK cells cultured for 24 h with and without IGF-1 (control). The graphs show the average relative frequency of all perforin + , CD107a + or Granzyme B + dNK cells as above. ( d ) Relative PRF1 , GzmB and IFNG expression levels in purified human uterine dNK cells cultured for 24 h with IGF-1 at the indicated concentrations, as quantified by qRT–PCR. ( e ) Chromium-release assay using 51 Cr-labelled K562 cells co-cultured with untreated dNK cells (open squares) or dNK cells from the same preparation incubated for 24 h with IGF-1 (100 ng ml −1 ) in RPMI medium 1640 plus 10% fetal calf serum (filled squares) at various effector-to-target (E:T) ratios. ( f ) YT and primary dNK cells were deprived of serum for 4 h and were then stimulated with 100 ng ml −1 IGF-1 for 0, 5, 15, 30 and 60 min, separately. The cells were washed by PBS and collected. The whole-cell extracts were prepared for western blotting to examine STAT3 and phosphorylation of STAT3. ( g , h ) The dNK cells were pretreated with WP1066 (100 μM) for 30 min or left untreated, followed by treatment with or without IGF-1 (100 ng ml −1 ) for 24 h. The presence of phospho-STAT3 was probed by western blot analysis ( g ), and perforin gene expression was quantified by qRT–PCR ( h ). Data are representative of three independent experiments (mean±s.e.m.). * P <0.05 and ** P <0.01 (Student’s t -test). ns, not significant. Full size image To determine whether IGF-1 induction of increased NK cytotoxic potential was restricted to the above in vitro differentiated NK experimental system, we assessed the role of IGF-1 in human uterine dNK cells, which possess reduced lytic activity. Similar to the in vitro differentiated NK system, a significant increase in the percentage of cells expressing perforin and CD107a was observed in dNK cells ( Fig. 2c ). The addition of exogenous IGF-1 (50–100 ng ml −1 ) caused a dose-dependent enhancement in the expression of the cytotoxic effector gene PRF1 , but no statistically significant differences could be detected for the mRNA levels of GzmB and IFNG in our experiments ( Fig. 2d ). Moreover, the incubation of dNK cells with K562 cells in an IGF-1-containing medium resulted in a substantial increase in the cytotoxic effector function of dNK cells ( Fig. 2e ). We also observed the surface expression of NKp30, NKp44, NKp46, NKG2D, CD16 and CD69 on dNK cells using flow-cytometric analysis. In contrast to what was observed with UCB/CD34 + NK cells, after incubation with 100 ng ml −1 IGF-1 for 24 or 48 h, the expression levels of the examined NK cell receptors (NKRs) in dNK cells were all augmented when compared with controls ( Supplementary Fig. S3 ), likely reflecting a discrepancy between the experimental systems in terms of the IGF-1 treatment time. We demonstrated above that exogenous IGF-1-enhanced NK cell cytotoxicity and also induced perforin gene expression in NK cells. In addition, it has been demonstrated that STAT3 is phosphorylized after cytokine stimulation and is a transcription factor for perforin in human NK cells [39] . To further understand the intracellular signalling mechanisms of IGF-1-stimulated NK cells, we evaluated the kinetics of IGF-1-mediated STAT3 phosphorylation in human NK cell line YT cells and primary dNK cells. As shown in Fig. 2f , whole-cell extracts from IGF-1-treated NK cells demonstrated activation of STAT3. Furthermore, WP1066 (a specific inhibitor of STAT3) dramatically attenuated IGF-1-stimulated STAT3 activity ( Fig. 2g ). Interestingly, the attenuation of STAT3 activation correlated with attenuation of perforin expression ( Fig. 2h ). Moreover, NK cells transfected with small interfering RNA (siRNA) against PRF1 showed dramatic decreases in PRF1 expression, coupled with downregulated NK cell cytotoxicity (data not shown), suggesting that perforin is an essential factor for determining NK cell killing capacity. Taken together, these results demonstrated that IGF-1 might promote perforin-mediated cytotoxicity via cell signalling through the STAT3 pathways in human NK cells. Endogenous IGF-1 is critical to human NK cell cytotoxicity Protein array data have shown IGF-1 to be preferentially produced by CD56 dim NK cells relative to CD56 bright NK cells [22] , suggesting that human NK cells have the ability to produce IGF-1. To confirm IGF-1 expression in human primary NK cells, we activated purified human dNK and pNK cells with phorbol myristate acetate/ionomycin. After 4 h of stimulation, we assayed for IGF-1 production in the culture supernatants. The dNK cells had a lower production of IGF-1 compared with pNK cells ( Fig. 3a ). We also examined IGF-1R expression in pNK and dNK cells and found similar IGF-1R expression levels in both cell types ( Fig. 3b ). Given the finding that dNK cells produced less IGF-1 ( Fig. 3a ) and that dNK cells had low perforin expression and displayed reduced lytic activity ( Fig. 3c ), we hypothesized that the ability to produce autocrine IGF-1 may be important for NK cell cytotoxicity. To confirm the above hypothesis, we performed several experiments. We knocked down IGF-1 expression and assayed the mRNA levels of PRF1 , GzmB and IFNG in human NK cells. As shown in Fig. 3e , knockdown of IGF-1 in YT cells resulted in the downregulation of PRF1 gene expression. Next, we assessed the requirement of IGF-1 for the induction of cytotoxicity in human primary NK cells. The pNK cells display high lytic activity; however, that activity was largely reduced when pNK cells were treated with an IGF-1-neutralizing antibody ( Fig. 3f ), indicating that human NK cell cytotoxicity is dependent on endogenous IGF-1. In addition, we determined that dNK cells from human patients who underwent spontaneous abortions had higher expression of IGF-1 ( Fig. 3g ), higher cytotoxic activity and increased perforin expression when compared with dNK cells from age-matched healthy controls ( Fig. 3h–j ). In sum, these data suggest that endogenous IGF-1 is critical to the cytotoxic activity of human NK cells. 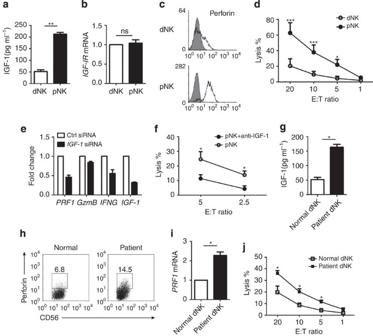Figure 3: Endogenous IGF-1 is critical for the cytotoxic activity of human NK cells. (a) IGF-1 levels in the supernatants of purified human pNK and dNK cells stimulatedin vitrowith phorbol myristate acetate/ionomycin, as assessed by ELISA at 4 h of culture. (b)IGF-1Rexpression in purified pNK and dNK cells, as quantified by quantitative reverse transcription PCR (qRT–PCR). (c) Flow cytometry for perforin expression in freshly isolated pNK and dNK cells. The grey histogram represents the isotype-matched negative controls. (d)51Cr release assays evaluating the lytic activity of dNK and pNK cells on the K562 target cell lines. (e)PRF1,GzmB,IFNGandIGF-1expression in YT cell lines transfected withIGF-1siRNA or control siRNA, as quantified by qRT–PCR. Data are representative of three independent experiments with similar results. (f) Chromium-release assays evaluating the lytic activity of pNK cells on the K562 target cell lines in the absence or presence of IGF-1-neutralizing antibody (anti-IGF-1). (g–j) ELISA of IGF-1 in culture supernatants (g), intracellular staining of perforin (h), qRT–PCR analysis ofPRF1expression (i) and the cytotoxic activity (j) of dNK cells from human patients with spontaneous abortions or age-matched healthy controls. Data are from three independent experiments (mean±s.e.m.) (d–f,j) or from four samples (mean±s.d.) (a,b,g,i) or one experiment representative of three independent experiments with similar results (c,h). *P<0.05,**P<0.01 and***P<0.005 (Student’st-test). E:T, effector-to-target. Figure 3: Endogenous IGF-1 is critical for the cytotoxic activity of human NK cells. ( a ) IGF-1 levels in the supernatants of purified human pNK and dNK cells stimulated in vitro with phorbol myristate acetate/ionomycin, as assessed by ELISA at 4 h of culture. ( b ) IGF-1R expression in purified pNK and dNK cells, as quantified by quantitative reverse transcription PCR (qRT–PCR). ( c ) Flow cytometry for perforin expression in freshly isolated pNK and dNK cells. The grey histogram represents the isotype-matched negative controls. ( d ) 51 Cr release assays evaluating the lytic activity of dNK and pNK cells on the K562 target cell lines. ( e ) PRF1 , GzmB , IFNG and IGF-1 expression in YT cell lines transfected with IGF-1 siRNA or control siRNA, as quantified by qRT–PCR. Data are representative of three independent experiments with similar results. ( f ) Chromium-release assays evaluating the lytic activity of pNK cells on the K562 target cell lines in the absence or presence of IGF-1-neutralizing antibody (anti-IGF-1). ( g – j ) ELISA of IGF-1 in culture supernatants ( g ), intracellular staining of perforin ( h ), qRT–PCR analysis of PRF1 expression ( i ) and the cytotoxic activity ( j ) of dNK cells from human patients with spontaneous abortions or age-matched healthy controls. Data are from three independent experiments (mean±s.e.m.) ( d – f , j ) or from four samples (mean±s.d.) ( a , b , g , i ) or one experiment representative of three independent experiments with similar results ( c , h ). * P <0.05, ** P <0.01 and *** P <0.005 (Student’s t -test). E:T, effector-to-target. Full size image IGF-1 expression is regulated by hsa-miR-483-3p Although the changing expression of IGF-1 evidently contributed to higher cytotoxicity in human NK cells, it was unclear what underlying mechanisms controlled IGF-1 expression. The miRNA, which controls gene expression post-transcriptionally by binding the 3′ UTR of target mRNA, has emerged as an important component in the differentiation and function of cells involved in the immune response [40] . Therefore, we hypothesized that the 3′ UTR of the IGF-1 gene may be targeted for downregulation by miRNAs in NK cells, leading to attenuation of their cytotoxicity. To test our hypothesis, we initially assessed miRNA expression in human primary lymphocytes with miRNA microarray. We purified T, NKT and pNK cells from PBMCs, cNK cells from cord blood mononuclear cells and dNK cells from uterine deciduas from healthy donors using flow-cytometry sorting. Next, we searched for miRNAs that were preferentially expressed in select human lymphocytes subsets and found nine miRNAs to have subset-specific expression ( Fig. 4a ). We focused on miR-483-3p because it had the greatest difference in expression in dNK cells versus the other subsets ( Fig. 4b ), and more importantly, because it was predicted by TargetScan to target the IGF-1 gene [41] ( Supplementary Fig. S4 , Fig. 4d ). Thus, miR-483-3p is a strong candidate repressor of the IGF-1 gene. According to the TargetScan algorithm, we identified two putative binding sites in the IGF-1 3′ UTR. To investigate whether one or both putative binding sites were functional, we cloned fragments of 98 and 96 bp of the human IGF-1 3′ UTR mRNA (NM_ 000618) containing the two putative miRNA-binding sites into the psiCHEK-2 vector ( Supplementary Fig. S4b ) and transfected these constructed vectors into HEK293 cells along with synthetic mature miR-483-3p double-stranded RNA (miR-483-3p mimic, miR-483-3p) or a control miRNA (miR-C) with a scrambled sequence. After normalization of the Renilla luciferase signal to the firefly luciferase signal, miR-483-3p induced a significant decrease in the normalized luciferase activity of the vector containing the putative miRNA-binding site 2 compared with control, whereas it had no inhibitory effect on the activity of binding site 1 ( Fig. 4e ). In addition, deletion of the miR-483-3p-responsive elements in binding site 2 of the IGF-1 3′ UTR resulted in abrogation of the inhibitory effect of miR-483-3p, indicating that only site 2 was functional ( Fig. 4f ). Next, we tested the ability of miR-483-3p to regulate endogenous IGF-1 expression. Our results demonstrated that the mRNA and protein levels of IGF-1 were both decreased in A549 cells transfected with the miR-483-3p mimic ( Fig. 4g ). We further assessed the ability of endogenous miR-483-3p to regulate IGF-1 expression in human primary NK cells. In comparison with the miRNA control, the mRNA and protein levels of IGF-1 were upregulated when miR-483-3p was knocked down with anti-miR-483-3p in human dNK cells ( Fig. 4i ). 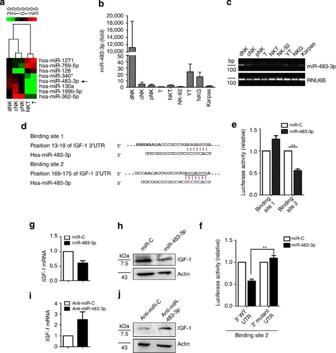Figure 4: Direct targeting of the 3′ UTR ofIGF-1mRNA by miR-483-3p. (a) Heatmap comparing various human lymphocyte subsets. (b) Quantitative reverse transcription PCR (qRT–PCR) analysis of miR-483-3p expression in various lymphocyte subsets. (c) The products of qRT–PCR inbdetected by agarose electrophoresis. (d) Predicted interaction between miR-483-3p and the two putative binding sites in the IGF-1 3′ UTR. (e) Dual-luciferase assay of HEK293T cells transfected with luciferase constructs containing the two putative miR-483-3p-binding sites (binding site 1 or binding site 2) together with synthetic mature miR-483-3p (miR-483-3p) or a synthetic control miRNA with a scrambled sequence (miR-C).**P<0.01, relative to miR-C control (Student’st-test). (f) Dual-luciferase assay (as ine) of HEK293T cells transfected with luciferase constructs containing the wild-type 3′ UTR (3′ WT UTR) or a mutated 3′ UTR (3′ mutant UTR) (with deletion of the miR-483-3p-responsive element) fromIGF-1, plus miRNA (as ine).**P<0.01 (Student’st-test). (g,h) qRT–PCR analysis (g) and immunoblot analysis (h) of the expression of IGF-1 in A549 cells transfected with synthetic mature miR-483-3p (miR-483-3p) or a synthetic control miRNA with scrambled sequence (miR-C). (i,j) qRT–PCR analysis (i) and immunoblot analysis (j) of the expression of IGF-1 in dNK cells transfected with the synthetic miR-483-3p inhibitor (anti-miR-483-3p) or a synthetic control miRNA (anti-miR-C). Data are from three independent experiments with similar results. E:T, effector-to-target. Figure 4: Direct targeting of the 3′ UTR of IGF-1 mRNA by miR-483-3p. ( a ) Heatmap comparing various human lymphocyte subsets. ( b ) Quantitative reverse transcription PCR (qRT–PCR) analysis of miR-483-3p expression in various lymphocyte subsets. ( c ) The products of qRT–PCR in b detected by agarose electrophoresis. ( d ) Predicted interaction between miR-483-3p and the two putative binding sites in the IGF-1 3′ UTR. ( e ) Dual-luciferase assay of HEK293T cells transfected with luciferase constructs containing the two putative miR-483-3p-binding sites (binding site 1 or binding site 2) together with synthetic mature miR-483-3p (miR-483-3p) or a synthetic control miRNA with a scrambled sequence (miR-C). ** P <0.01, relative to miR-C control (Student’s t -test). ( f ) Dual-luciferase assay (as in e ) of HEK293T cells transfected with luciferase constructs containing the wild-type 3′ UTR (3′ WT UTR) or a mutated 3′ UTR (3′ mutant UTR) (with deletion of the miR-483-3p-responsive element) from IGF-1 , plus miRNA (as in e ). ** P <0.01 (Student’s t -test). ( g , h ) qRT–PCR analysis ( g ) and immunoblot analysis ( h ) of the expression of IGF-1 in A549 cells transfected with synthetic mature miR-483-3p (miR-483-3p) or a synthetic control miRNA with scrambled sequence (miR-C). ( i , j ) qRT–PCR analysis ( i ) and immunoblot analysis ( j ) of the expression of IGF-1 in dNK cells transfected with the synthetic miR-483-3p inhibitor (anti-miR-483-3p) or a synthetic control miRNA (anti-miR-C). Data are from three independent experiments with similar results. E:T, effector-to-target. Full size image miR-483-3p upregulation reduces human NK cell cytotoxicity Given the finding that endogenous IGF-1 is critical to the cytotoxic activity of human NK cells and that miR-483-3p can regulate IGF-1 expression, we hypothesized that miR-483-3p may regulate NK cell cytotoxic activity, at least in part, through IGF-1. To test our hypothesis, we studied the functional role of miR-483-3p in modulating NK cell cytotoxic activity using a gain-of-function approach. YT cells transfected with the miR-483-3p mimic expressed substantially more miR-483-3p but less PRF1 gene than did cells transfected with a negative-control miRNA ( Fig. 5a ). Another human NK cell line, NK-92 cells also exhibited decreased PRF1 mRNA levels and concomitantly reduced NK cell cytotoxic activity after miR-483-3p expression ( Fig. 5c–e ). 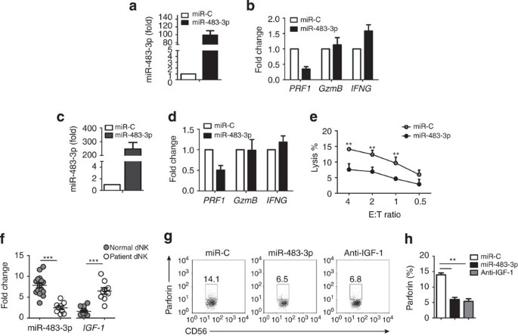Figure 5: Overexpression of miR-483-3p inhibits human NK cell cytotoxic potential. (a–d) qRT–PCR assay of miR-483-3p (a,c) andPRF1,GzmBandIFNG(b,d) in YT cells (a,b) and in NK-92 cells (c,d) transfected with synthetic mature miR-483-3p (miR-483-3p) or a synthetic control miRNA with a scrambled sequence (miR-C). (e) Chromium-release assays evaluating the lytic activity of the NK-92 cells in (c,d). (f) Quantitative PCR analysis of miR-483-3p andIGF-1in dNK cells from human patients with spontaneous abortion or age-matched healthy controls. (g) Flow cytometry of the intracellular expression of perforin in purified dNK cells from human patients with spontaneous abortion transfected by nucleofection with synthetic mature miR-483-3p (miR-483-3p) or a synthetic control miRNA with a scrambled sequence (miR-C), or treated with IGF-1-neutralizing antibody (anti-IGF-1). (h) The average relative frequency of perforin+dNK cells ing(average of three replicates). Data are representative of three independent experiments (mean±s.e.m.).**P<0.01 and***P<0.005 (Student’st-test). E:T, effector-to-target. Figure 5: Overexpression of miR-483-3p inhibits human NK cell cytotoxic potential. ( a – d ) qRT–PCR assay of miR-483-3p ( a , c ) and PRF1 , GzmB and IFNG ( b , d ) in YT cells ( a , b ) and in NK-92 cells ( c , d ) transfected with synthetic mature miR-483-3p (miR-483-3p) or a synthetic control miRNA with a scrambled sequence (miR-C). ( e ) Chromium-release assays evaluating the lytic activity of the NK-92 cells in ( c , d ). ( f ) Quantitative PCR analysis of miR-483-3p and IGF-1 in dNK cells from human patients with spontaneous abortion or age-matched healthy controls. ( g ) Flow cytometry of the intracellular expression of perforin in purified dNK cells from human patients with spontaneous abortion transfected by nucleofection with synthetic mature miR-483-3p (miR-483-3p) or a synthetic control miRNA with a scrambled sequence (miR-C), or treated with IGF-1-neutralizing antibody (anti-IGF-1). ( h ) The average relative frequency of perforin + dNK cells in g (average of three replicates). Data are representative of three independent experiments (mean±s.e.m.). ** P <0.01 and *** P <0.005 (Student’s t -test). E:T, effector-to-target. Full size image We next evaluate miR-483-3p expression in dNK cells from patients who underwent spontaneous abortions on the basis of our findings of higher perforin expression and cytotoxicity in these cells ( Fig. 3h–j ). Strikingly, these cells had significantly lower expression of miR-483-3p, which inversely correlated with the expression of IGF-1 when compared with dNK cells from age-matched healthy controls ( Fig. 5f ), suggesting that miR-483-3p may function as a modulator of IGF-1 and perforin expression in human dNK cells. To confirm this hypothesis, we next transfected dNK cells from patients who underwent spontaneous abortions with the miR-483-3p mimic. The overexpression of miR-483-3p resulted in significantly reduced perforin expression; a similar decrease was observed in dNK cells treated with IGF-1-neutralizing antibody (anti-IGF-1) ( Fig. 5g ). Based on all of the above results, we conclude that miR-483-3p inhibits perforin expression and cytotoxicity in human NK cells by directly targeting IGF-1. Knockdown of miR-483-3p enhances human NK cell cytotoxicity Next, we examined the effect of miR-483-3p loss-of-function on the cytotoxic activity of human NK cells. The dNK cells showed a dramatic increase in their cytotoxic activity when transfected with a miR-483-3p inhibitor (anti-miR-483-3p) ( Fig. 6a ), in addition to upregulated perforin expression and CD107a release ( Fig. 6b–d ). The acquisition of cytotoxic function by NK cells is related to the appearance of a series of receptors on the effector cells. To investigate whether the increased cytotoxic activity of dNK cells may be attributable to differences in NKRs, we examined the expression of NKp30, NKp44, NKp46 and NKG2D in dNK cells transfected with miR-483-3p inhibitor or a control miRNA. All of the above NKRs in dNK cells were upregulated after transfection with the miR-483-3p inhibitor relative to control ( Supplementary Fig. S5 ). Similar to dNK cells, miR-483-3p inhibitor-transfected NK cells derived from UCB/CD34 + HSCs demonstrated upregulation of perforin and CD107a ( Supplementary Fig. S6 ). 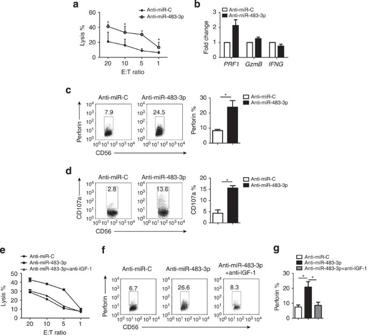Figure 6: Inhibition of miR-483-3p acts by IGF-1 to enhance the cytotoxic activity of human NK cells. (a) Chromium-release assays evaluating the lytic activity of dNK cells transfected with synthetic miR-483-3p inhibitor (anti-miR-483-3p) or a synthetic control miRNA (anti-miR-C). (b) qRT–PCR analysis of the expression ofPRF1,GzmBandIFNGin purified dNK cells ina. (c,d) Flow cytometry for perforin (c) and CD107a (d) expression on the purified dNK cells in (a). The graphs show the average relative frequency of perforin+or CD107a+cells as above. (e,f) Chromium-release assays evaluating the lytic activity (e) and flow-cytometry analysis for perforin expression (f) of purified dNK cells transfected with the miR-483-3p inhibitor (anti-miR-483-3p) in the presence or absence of IGF-1-neutralizing antibody (anti-IGF-1). (g) The average relative frequency of perforin+dNK cells ing. *P<0.05 and**P<0.01 versus control (Student’st-test). Data are from three independent experiments (mean±s.e.m.). E:T, effector-to-target. Figure 6: Inhibition of miR-483-3p acts by IGF-1 to enhance the cytotoxic activity of human NK cells. ( a ) Chromium-release assays evaluating the lytic activity of dNK cells transfected with synthetic miR-483-3p inhibitor (anti-miR-483-3p) or a synthetic control miRNA (anti-miR-C). ( b ) qRT–PCR analysis of the expression of PRF1 , GzmB and IFNG in purified dNK cells in a . ( c , d ) Flow cytometry for perforin ( c ) and CD107a ( d ) expression on the purified dNK cells in ( a ). The graphs show the average relative frequency of perforin + or CD107a + cells as above. ( e , f ) Chromium-release assays evaluating the lytic activity ( e ) and flow-cytometry analysis for perforin expression ( f ) of purified dNK cells transfected with the miR-483-3p inhibitor (anti-miR-483-3p) in the presence or absence of IGF-1-neutralizing antibody (anti-IGF-1). ( g ) The average relative frequency of perforin + dNK cells in g . * P <0.05 and ** P <0.01 versus control (Student’s t -test). Data are from three independent experiments (mean±s.e.m.). E:T, effector-to-target. Full size image To test the hypothesis that increased IGF-1 levels may mediate the effects of anti-miR-483-3p, we added IGF-1-neutralizing antibody (anti-IGF-1) to the anti-miR-483-3p-transfected dNK cell culture to neutralize the expression of IGF-1. Indeed, IGF-1-neutralizing antibody reversed the increases in dNK cell cytotoxic activity ( Fig. 6e ) and perforin expression ( Fig. 6f ). We conclude that miR-483-3p acts through IGF-1 to regulate the cytotoxic activity of human NK cells. Previous studies have demonstrated that IGF-1 can regulate hematopoiesis and diverse functions of cells of the innate and acquired immune systems [17] , [18] , [19] , [20] , [21] . However, the detailed effects of IGF-1 on NK cell development and function remain largely unexplored. Our results show that IGF-1 promotes the development of NK cells derived from human CD34 + HSCs and that endogenous IGF-1 regulated by miR-483-3p is critical to NK cell activity. We reveal that IGF-1 appears to send signals for both differentiation and proliferation in the course of NK cell maturation from human CD34 + cellular populations. The status of IRS-1 determines which of the above two signals of IGF-1 predominates in cultured CD34 + cells. Moreover, the mechanism by which IGF-1 promotes the production of NK cell populations is also associated with upregulated mRNA signals for NFIL3 ( E4BP4 ) and ID2 , which are critical transcription factors for NK cell development [33] , [42] . Previous studies have cited the positive effect of IGF-1 on human pNK cell cytotoxicity [21] , [43] . However, the exact regulatory mechanism of IGF-1 on NK cell function remains unclear. In the present study, we clearly show that IGF-1 stimulates the perforin gene and subsequent protein expression in HSC-derived NK cells and CD56 bright dNK cells. Moreover, IGF-1 induced a steep rise in the cytotoxic effector function of dNK cells. We further demonstrate that the STAT3 pathway is involved in the enhancement of NK cell cytotoxicity by IGF-1. An important component of the IGF system is represented by the IGF-2/IGF-2 receptor (IGF-2R) axis. In the present study, we also examined the effect of IGF-2 on human NK cells. Our results showed that NK cells express IGF-2R and that IGF-2 had no significant effect on NK cell phenotype or cytotoxic potential ( Supplementary Fig. S7 ).It is possible that, on human NK cells, although IGF-2 can exert its effects by binding to the IGF-2R, IGF-2 may also bind to the IGF-1R activating downstream effectors that are only partly similar to those induced by IGF-1. It has been indicated that IGF-1 has an important role in the promotion of mitogenesis and protection from apoptosis in many cell types [44] . In this study, we show that IGF-1 did increase proliferation but did not affect apoptosis in NK cells ( Supplementary Fig. S8 ). One possible explanation is that the effects of IGF-1 may simply vary depending on the doses or the experimental systems to which it is added. Previous studies have shown that exogenous IGF-1 has a positive effect on human pNK cell cytotoxicity. In this study, we identified a critical role for endogenous IGF-1 in the regulation of the cytotoxic activity of human NK cells. However, more precise analysis of NK cells in IGF-1 −/− or IGF-1R −/− mice will be required to entirely confirm the possibility of a key role for endogenous IGF-1 in NK cell cytotoxicity. Previous reports have shown that miR-483-3p functions as an oncogene by modulating multiple target genes in various human cancers [45] .In the present study, we reveal that miR-483-3p functions as a critical regulator of human NK cell cytotoxicity by directly targeting IGF-1. We reported that dNK cells from patients who underwent spontaneous abortions showed lower miR-483-3p expression, which correlated well with increased IGF-1 production, perforin expression and cytotoxic activity when compared with dNK cells from healthy controls. It has been reported that IGF-1 overexpression can cause fetal loss during placentation in mice; these high levels of IGF-1 could directly alter the characteristics and functions of the uterine NK cells [46] . Our histological analysis data also show that IGF-1 expression is higher in decidual tissues from patients with spontaneous abortions than in tissues from healthy controls in vivo ( Supplementary Fig. S9 ). Although it is tempting to speculate that it is endogenous IGF-1 that is critical for NK cell cytotoxicity, we cannot rule out the possibility that there is some contribution of exogenous IGF-1 from circumstances in vivo . However, the in vitro data indicate that this cytotoxicity and the perforin expression levels in NK cells appear to be dependent upon endogenous IGF-1 and miR-483-3p expression, given that they can be inhibited by either IGF-1-neutralizing antibody or miR-483-3p overexpression. In conclusion, the findings presented here identify a previously unrecognized role for IGF-1 in the positive regulation of human NK cell development and cytotoxicity. Moreover, the finding that endogenous IGF-1 regulation by miR-483-3p is critical for human NK cell cytotoxic activity provides new mechanistic insights into the biology of human NK cells. In terms of the importance of NK cells in immunotherapy, such information might present new opportunities for boosting or limiting NK cell cytotoxicity therapeutically. Samples All decidual samples from patients undergoing elective abortion were collected at Hefei Maternity and Child Care Hospital. Clinical characteristics were listed in Supplementary Table S1 . Cord blood samples from the umbilical cords of the placentas of normal, full-term, non-stressed newborns of consenting mothers were also collected at Hefei Maternity and Child Care Hospital. Adult peripheral blood samples were obtained from healthy donors at Hefei Blood Bank. All blood samples were obtained after donor informed consent and approval by the Ethics Committee of the University of Science and Technology of China. Reagents and antibodies Recombinant human SCF, rhFlt3-L, rhIL-15 and rhIGF-1 were from PeproTech, USA. The neutralizing antibody against IGF-1 (human IGF-1 antibody, goat IgG) was from R&D Systems, and the anti-IGF-1 mouse monoclonal antibody was from Santa Cruz Biotechnology. Anti-IRS-1 rabbit polyclonal antibody, anti-phospho-STAT3 (Tyr705) rabbit monoclonal antibody and anti-STAT3 rabbit polyclonal antibody were obtained from Cell Signaling Technology. The STAT3 inhibitor WP1066 was obtained from Santa Cruz Biotechnology. The inhibitor was dissolved in dimethyl sulfoxide and was kept at −20 °C. The horseradish peroxidase-conjugated goat anti-mouse or goat anti-rabbit secondary antibody was purchased from Promega, and anti-β-actin was from Sigma. The following antibodies were from BD Pharmingen: anti-CD56 conjugated with Alexa-647; phycoerythrin (PE)-Cy5-conjugated anti-CD3 monoclonal antibodies; anti-CD16; anti-Granzyme B conjugated with fluorescein isothiocyanate (FITC); and PE-conjugated anti-CD34, anti-NKp30, anti-NKp44, anti-NKp46, anti-NKG2D, anti-CD69, anti-perforin and anti-CD107a. Isotype-matched negative-control antibodies labelled with FITC, PE, PE-Cy5 or Alexa-647 were all from BD Pharmingen. Cell preparation and purification The cells were processed within 4 h of collection. Blood samples were diluted 1:2 in PBS. Mononuclear cells were isolated by Ficoll-Hypaque centrifugation using standard procedures. In some experiments, CD34 + or CD56 + NK cells were isolated from cord blood mononuclear cells with the MACS isolation system according to the manufacturer’s instructions (Miltenyi Biotec). NK (CD3 − CD56 + ), NKT (CD3 + CD56 + ) and T (CD3 + CD56 − ) lymphocyte subsets were purified from PBMCs by sorting on a FACS Aria (BD) according to various combinations of surface markers. The dNK cells were isolated from decidual samples as previously described [12] . Cell purity was >90% by post-FACS analysis. The human NK-92 immortal cell line was grown in α-MEM (Life Technologies) supplemented with 15% heat-inactivated fetal bovine serum, 15% horse serum and 100 U ml −1 IL-2 and streptomycin/penicillin. The human YT immortal cell line and human K562 erythroleukemia cells were grown in RPMI 1640 medium (Gibco BRL) supplemented with 10% fetal bovine serum (Hyclone) and streptomycin/penicillin. Generation of human UCB/CD34 + cell-derived NK cells Human UCB/CD34 + cell-derived NK cells were prepared according to a modified protocol originally described previously [47] . Briefly, freshly isolated CD34 + cells (1 × 10 5 cells per well) were cultured with GMP Serum-free Stem Cell Growth Medium (CellGro/CellGenix) supplemented with 30 ng ml −1 SCF and 50 ng ml −1 Flt3-L (PeproTech). IL-15 (50 ng ml −1 ; PeproTech) and/or IGF-1 (100 ng ml −1 ; PeproTech) were added to SCF/Flt3-L-containing cultures as specified in the figure legends. The plates were incubated for 4 weeks at 37 °C in a humidified atmosphere with 5% CO 2 . Half of the medium volume was replaced with fresh medium and cytokines twice every week. RNA Isolation and Real-Time PCR Analysis Total RNA was isolated with TRIzol Reagent (Invitrogen). RNA was then reverse transcribed using Moloney murine leukemia virus reverse transcriptase (Invitrogen) and random primers (Roche). The cDNA was amplified with specific primers and Power SYBR Green PCR Master Mix (Applied Biosystems). The GAPDH mRNA level was used as an internal normalization control. The sequences of the primers used were as follows: NFIL3 , 5′-CTGCTTTAACGGAAGTGTCAGA-3′(forward), 5′-TTCCTCCGACATGCAGAAGAT-3′(reverse); ID2 , 5′-AGTCCCGTGAGGTCCGTTAG-3′ (forward), 5′-AGTCGTTCATGTTGTATAGCAGG-3′(reverse); PRF1 , 5′-CGCCTACCTCAGGCTTATCTC-3′ (forward), 5′-CCTCGACAGTCAGGCAGTC-3′ (reverse); GzmB , 5′-CCCTGGGAAAACACTCACACA-3′(forward), 5′-CACAACTCAATGGTACTGTCGT-3′ (reverse); IFNG , 5′-TCGGTAACTGACTTGAATGTCCA-3′(forward), 5′-TCCTTTTTCGCTTCCCTGTTTT-3′ (reverse); IGF-1 , 5′-AGGAAGTACATTTGAAGAACGCAAGT-3′ (forward), 5′-CCTGCGGTGGCATGTCA-3′ (reverse); IGF-1 R , 5′-AAAATGCTGACCTCTGTTACCTC-3′(forward), 5′-GCTTATTCCCCACAATGTAGTT-3′(reverse); IRS-1 , 5′-CTGCACAACCGTGCTAAGG-3′ (forward), 5′-CGTCACCGTAGCTCAAGTCC-3′ (reverse); and GAPDH , 5′-ATGGGGAAGGTGAAGGTCG-3′ (forward), 5′-GGGGTCATTGATGGCAACAATA-3′ (reverse). For miRNA analysis, real-time PCR was carried out according to the manufacturer’s instructions (Qiagen; miScript Reverse Transcription kit, catalogue no. 218060; miScript Primer Assay for hsa-miR-483-3p, catalogue no. MS00009751 and miScript SYBR Green PCR kit, catalogue no. 218073). Then, miRNA was normalized to the small nucleolar RNA RNU6B (primer assay, catalogue no. MS00014000). Enzyme-linked immunosorbent assay IGF-1 in culture supernatants was quantified with an enzyme-linked immunosorbent assay (ELISA) kit (Boster). BrdU cell-proliferation assay The rate of DNA synthesis was determined from the incorporation of BrdU into cells (BrdU Cell Proliferation ELISA kit; MAi Bio Co.) according to the manufacturer’s instruction. Briefly, cells were seeded at 2 × 10 5 cells per well on a 96-well microplate and cultured with or without IGF-1(100 ng ml −1 ) for 24 h to allow BrdU incorporation. After fixation, the cells were incubated with anti-BrdU antibody for 2 h, followed by HRP-conjugated goat anti-mouse IgG. Then, 100 μl of substrate (tetramethylbenzidine) was added to each well after washing and incubated at room temperature for 30 min. The absorbance at dual wave lengths of 450–550 nm was determined using the microplate reader. Dual-luciferase assay HEK293T cells were transfected with 10 ng each of psiCHECK-2 construct along with 15 pmol of the miR-483-3p mimic or an identical amount of the control mimic with Lipofectamine 2000 (Invitrogen). After 48 h, the cells were lysed, and the firefly and Renilla luciferase activities were measured with the Dual-Luciferase Reporter Assay System (Promega). Each fragment containing the putative miRNA-binding sites was cloned in psiCHECK-2 immediately downstream of the gene encoding renilla luciferase. The results are presented as the ratio of Renilla luciferase activity to firefly luciferase activity. Nucleofection Pre-made siRNAs against human IGF-1, miRNA mimics and miRNA hairpin inhibitors were purchased from GenePharma. An Amaxa Cell Line Nucleofector Kit R (VCA-1001) was used for transfection of NK-92 cells, and an Amaxa Cell Line Nucleofector Kit V (VCA-1003) was used for YT cells. An Amaxa Human NK Cell Nucleofector Kit (VPA-1005) was used for transfection of human primary NK cells, and an Amaxa Human CD34 + Cell Nucleofector Kit (VPA-1003) was used for transfection of human CD34 + -derived NK cells. Cells were plated in complete medium and subjected to IB analysis, real-time quantitative PCR, FACS analysis or standard 51 Cr release. Immunoblot analysis Cells were collected and lysed in RIPA buffer supplemented with protease inhibitors (Pierce). After centrifugation at 20 000 g for 20 min to remove cell debris, the pellet was discarded. The protein concentration in the supernatant was determined by bicinchoninic acid assay (BCA) (Pierce). Equal amounts of protein from cell lysates were separated by 4–20% SDS–PAGE. Gels were transferred to PVDF (polyvinylidene difluoride) membranes followed by probing with primary antibody solutions (1:200 for IGF-1, 1:1000 for IRS-1, phospho-STAT3 and STAT3, and 1:500 for actin) overnight at 4 °C. The membrane was then incubated with appropriate horseradish peroxidase-conjugated secondary antibodies (1:5000). Immunoreactive protein bands were developed by chemiluminescence autoradiography. NK cell degranulation and cytotoxicity NK cell degranulation was measured by flow cytometry as described with slight modifications [38] . Briefly, 2 × 10 5 human NK cells and 2 × 10 5 cells of the erythroleukemia cell line K562 (American Type Culture Collection) were mixed by gentle pipetting, spun down for 1 min at 1000, r.p.m. and incubated for 2 h at 37 °C in 200 μl of media as indicated. NK cells were then stained with an Alexa-647-labelled anti-CD56-Ab, and degranulation was detected with a PE-labelled anti-CD107a-Ab (all Abs from BD Biosciences). The cytotoxic activity of cultured cells was determined in a standard 4-h 51 Cr release assay against K562. Briefly, K562 cells were labelled with 200 μCi of sodium chromate ( 51 Cr) (Perkin-Elmer) per 10 6 cells for 1 h at 37 °C. Effector cells were incubated with K562 in 96-well round bottom plates for 4 h at 37 °C and 5% CO 2 . The percentage of specific lysis was calculated from the formula as follows: (experimental release−spontaneous release)/(maximum release−spontaneous release) × 100%. Statistics A two-tailed Student’s t -test was used for statistical comparison of two groups, and P- values ≤0.05 were taken as statistically significant. How to cite this article: Ni, F. et al. IGF-1 promotes the development and cytotoxic activity of human NK cells. Nat. Commun. 4:1479 doi: 10.1038/ncomms2484 (2013).